Reply to: Assessing the precision of morphogen gradients in neural tube development 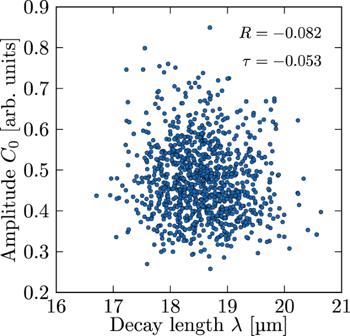Fig. 1: Absence of correlation between gradient amplitude and decay length in a cell-based model with independent cell-to-cell molecular noise. Data fromn= 1000 simulated gradients obtained with independent noise between individual cells in all three kinetic parameters, CVp,d,D= 0.3. See1for method details. Pearson’s R = −0.082 (p= 0.010), Kendall’s τ = −0.053 (p= 0.012). Further information on research design is available in the Nature Portfolio Reporting Summary linked to this article.